Climate change drives microevolution in a wild bird To ensure long-term persistence, organisms must adapt to climate change, but an evolutionary response to a quantified selection pressure driven by climate change has not been empirically demonstrated in a wild population. Here, we show that pheomelanin-based plumage colouration in tawny owls is a highly heritable trait, consistent with a simple Mendelian pattern of brown (dark) dominance over grey (pale). We show that strong viability selection against the brown morph occurs, but only under snow-rich winters. As winter conditions became milder in the last decades, selection against the brown morph diminished. Concurrent with this reduced selection, the frequency of brown morphs increased rapidly in our study population during the last 28 years and nationwide during the last 48 years. Hence, we show the first evidence that recent climate change alters natural selection in a wild population leading to a microevolutionary response, which demonstrates the ability of wild populations to evolve in response to climate change. Global climate warming changes the environment of most organisms and is expected to lead to a change in selection pressures with microevolutionary consequences that allow the adaptation of organisms to this new environment and thereby long-term population persistence [1] . Although such adaptation to new environmental conditions created by climate change is expected in wild-animal populations [2] , solid evidence for a microevolutionary (that is, genetic) response to climate change is rare [3] . Microevolution in response to climate change has been demonstrated in invertebrate populations [4] , [5] , but these studies lack information on the mechanisms and selective factors linking particular genotypes to climate. Other studies have found selection on heritable phenotypic traits correlated with climate change, but do not report any genetic change in the population [3] or the role of environmental factors exceed those of selection and lead to unpredicted phenotypic changes [6] . The relative role of evolutionary versus ecological response in relation to climate change is still largely unexplored [6] , [7] , [8] . Furthermore, there is a noticeable absence of empirical studies addressing whether climate change actually has the potential to drive changes in selection and thereby cause microevolution [9] . Systems with genetically based colour polymorphism have been used in classic studies of microevolution in wild populations [10] , [11] , because they allow assessment of genotypes by censusing the frequency of colour morphs. Colour polymorphism is thought to have evolved and to be maintained by morph-specific sensitivity to environmental conditions [12] , [13] , [14] , and colour polymorphism often has a relatively simple genetic basis [15] , [16] . Hence, such systems should be highly suitable for studying the microevolutionary capacity of wild populations to track environmental change. In this study, we explore the links between climate change and alteration of the selective regime on a highly heritable phenotypic trait, plumage colouration in the tawny owl ( Strix aluco ), a common bird of prey throughout the temperate regions of Europe. In tawny owls, plumage colouration is determined by the degree of reddish-brown pheomelanin pigmentation deposited in their plumage [17] . This colouration is independent of age and sex, and is highly heritable [18] . The frequency distribution of colouration (scored on an ordinal scale) shows a bimodal distribution ( Fig. 1 ), suggesting there are two basic morphs (termed grey and brown). Earlier work revealed that the brown tawny owl morph has reduced survival compared with the grey morph, resulting in lower lifetime reproductive success of the brown morph [18] . 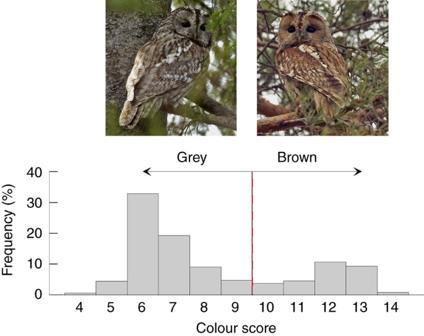Figure 1: Frequency distribution of tawny owl colouration in the study population. Colour scoring is based on scorings of brown pigmentation on four different parts of the plumage and ranges from 4 to 14 points in 491 individuals scored in 1978–2008. The frequency of colouration is bimodal and the two morphs can be classified into a grey and a brown morph at the cut point between scores 9 and 10. The cut point (red line) was determined visually as the lowest intermediate point between the two models18. A grey (left) and a brown (right) tawny owl colour morph are shown above the graph (photography courtesy of: Dick Forsman). Figure 1: Frequency distribution of tawny owl colouration in the study population. Colour scoring is based on scorings of brown pigmentation on four different parts of the plumage and ranges from 4 to 14 points in 491 individuals scored in 1978–2008. The frequency of colouration is bimodal and the two morphs can be classified into a grey and a brown morph at the cut point between scores 9 and 10. The cut point (red line) was determined visually as the lowest intermediate point between the two models [18] . A grey (left) and a brown (right) tawny owl colour morph are shown above the graph (photography courtesy of: Dick Forsman). Full size image In this study, we first use colour scores of parents and their offspring near fledging to demonstrate that a simple genetic architecture may underlie the two morphs. Second, we model the survival using capture–mark–recapture methodology of individual-based long-term data from 28 years in relation to climate conditions to show that selection against the brown morph is related to climate. Climate change has made winters increasingly milder during the last decades, and we show that selection against the brown morph disappeared accordingly. Last, we show that the proportion of the brown morph has increased dramatically over time. Thus, we have shown that climate change can influence selection demonstrating that climate change may influence evolution in wild populations. Heritability of colouration in tawny owls We colour scored all breeding tawny owls in our study population from 1978 onwards using a semi-continuous scale, which is based on scoring the degree of reddish-brown colouration in four different parts of the plumage. An individual's plumage colouration does not change throughout life (repeatability >90% (ref. 18 )). Because practically all male and female parents and their offspring have been individually marked in the study population since 1978, we can estimate the heritability using quantitative genetic methods [19] . We used a reduced pedigree, in which 167 individuals whose phenotype was measured and who had at least one relative with a measured phenotype in the pedigree were included. Extra-pair paternity is low in this species [20] , and we are thus confident in inferring relatedness on the basis of the social pedigree. Sex, age (1, 2, ≥3 years) and year of first breeding were tested as fixed effects, but were not significant, and were not included in the final models. This basic animal model based on the colouration scoring method revealed that plumage colouration was 79.8±13.8 (s.e.m. )% heritable, which is in accordance with previous high heritability estimates of colouration in tawny owls ranging from 72% using parent–offspring regression [18] and 93% in a cross-fostering experiment [17] . Such high heritability suggests that few genes have large effects on colouration of the phenotype. Inferring Mendelian genetics on nestlings and their parents Because the estimated heritability of colouration is high and the distribution of colour scores is bimodal ( Fig. 1 ), allowing the separation of two colour morphs, we tested whether a 'major gene' could be responsible for creating this pattern. We used data from 318 nestlings in 83 nests, which were colour scored as either brown or grey morph in years 2006–2009. Tawny owls mate random with respect to colour [18] . We contrasted three different models (see Supplementary Information ): two Mendelian models, in which plumage colour is assumed to be fully determined by one locus, where either the 'brown' allele is 100% dominant over the 'grey' allele or the other way around, and one additive genetic model (many genes of small, additive effect). The model assuming brown dominance ( Supplementary Table S1 ) produces a ratio of brown/grey phenotypes that almost exactly matches what is expected under this inheritance model in Hardy–Weinberg equilibrium (52.8% of offsprings are observed and 55.2% are expected to be brown, G 1 =0.308, P =0.58; Fig. 2 , Supplementary Table S2 ). Repeating the above, but assuming that the allele for grey morph is dominant over the allele for brown produces a poorer fit between observed and expected ratio of the offspring ( G 2 =12.98, P =0.0015; Fig. 2 ). There are more brown offspring observed than expected when assuming full dominance of the grey allele over brown. The purely additive model also fitted the data poorly. In this particular case, the colour scores of the adults were such that the additive model predicted that all offspring from monomorphic crosses were the same morph as the parents; thus, these crosses are not informative for testing. However, focusing on the heteromorphic (BxG) cross, it is clear that there are more offspring of the brown morph observed than expected also under the assumption of an additive genetic inheritance (G 1 =70.9, P <0.0001; Fig. 2 ). Alternative approaches for statistically comparing the observed and expected frequencies of morphs all provided the same conclusion ( Supplementary Information ). We thus conclude from the above exercises on the basis of comparing fledglings' morphs with their parents' morphs that we find evidence for genetic dominance of brown over grey, whereas dominance of grey and purely additive genetic effects are not supported by this data. Although this modelling is not exhaustive, it does show that the tawny owl phenotypic morph has a genetic architecture that relies on few genes with large effects, which is consistent with a Mendelian inheritance of colouration based on one locus with a 'brown' allele dominant over a 'grey' allele. 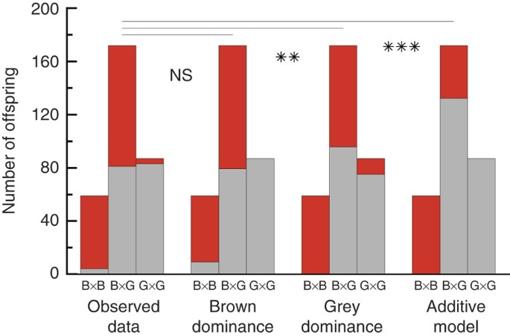Figure 2: Genetic models of inheritance of colouration. Number of brown (red bar) and grey (grey bar) offspring colour morphs produced by different combinations of parental colour morphs (B×B, B×G and G×G). The first columns show the observations in the field, second, third and fourth columns show the expected number of offspring colour morphs according to models with brown dominance, grey dominance and an additive genetic model, respectively. The lines above the bars show a G-test of association between models and their significance (NS:P=0.58, **P<0.002, ***P<0.0001). Figure 2: Genetic models of inheritance of colouration. Number of brown (red bar) and grey (grey bar) offspring colour morphs produced by different combinations of parental colour morphs (B×B, B×G and G×G). The first columns show the observations in the field, second, third and fourth columns show the expected number of offspring colour morphs according to models with brown dominance, grey dominance and an additive genetic model, respectively. The lines above the bars show a G-test of association between models and their significance (NS: P =0.58, ** P <0.002, *** P <0.0001). Full size image Climate change and survival of tawny owl colour morphs Several aspects of the environment have changed for tawny owls. Climate warming has led to milder winters, especially in subarctic regions [21] . Furthermore, the cyclic dynamics of voles—the staple food of tawny owls in Finland—has been fading and has become irregular in recent years [22] , [23] . We tested whether survival of tawny owl colour morphs are differently affected by such changes by applying capture–recapture modelling to the data from 1981 to 2008 ( N =466 individuals). We modelled survival probability of brown and grey adult breeding tawny owls in relation to over-winter prey abundance and snow depth and temperature during a period in winter that was critical for tawny owl survival (see Supplementary Information ). The results of the modelling showed that all four best models, which together received 99.4% of the support (QAICc weight), included an interaction where brown individuals had lower survival than grey ones as snow cover became deeper (col*snow, Table 1 ). Temperature (temp) was included in all four best models, which implies that low winter temperature decreases survival probability. There was also support for an interaction between colour morph and temperature (col*temp) indicating lower survival for brown individuals compared with grey ones in cold temperatures. Prey abundance in late autumn also explained some variation in survival, as the third ranked model included the effect of prey abundance (vole) and the fourth ranked model included an interaction between prey abundance and colour morph (col*vole). Recapture probability was not explained by variables prey abundance, temperature or snow depth as none of the models where recapture was constrained by these variables received any support. Table 1 Best five models explaining variation in survival of tawny owl colour morphs. Full size table Model averaging of all candidate models ( N =175) revealed that variation in snow depth explained most of the variation in survival of the colour morphs. In our case, 99.4% of support stems from the four best models ( Table 1 ) and the averaging can therefore be considered to mainly describe the common features included in these models (that is, colour morph–snow depth interaction). As snow depth increased, survival of the brown morph decreased more strongly than for the grey morph ( Fig. 3a ). Simultaneously, snow depth has decreased over time ( Fig. 3b ; linear model, year: b =−0.37±0.13, F 1,25 =8.49, P =0.007). As a consequence, there was a time trend in survival of the colour morphs from 1981–2008, in which survival of the grey morph was fairly stable across years, whereas survival of brown individuals improved dramatically towards the end of the time series ( Fig. 3c ). Thus, we provide evidence that climate-driven selection against the brown morph has decreased in recent years such that the survival propensity of the morphs have equalized in recent, mild winters. 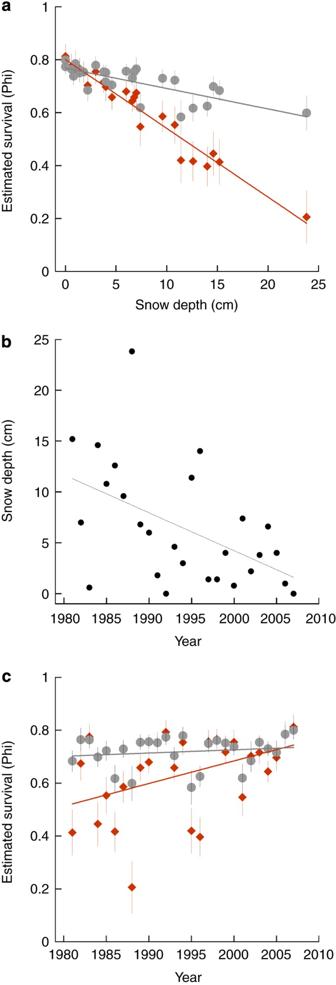Figure 3: Survival of grey and brown tawny owls in relation to changes in snow depth. Survival estimates are based on averaging all candidate capture–mark–recapture models considering the effects of food supply (vole abundance), average snow depth and average temperature during a critical period in winter (seeSupplementary Information). Climatic data are derived from the database of the Finnish Meteorological Institute. (a) Survival of brown and grey tawny owl colour morphs in relation to snow depth. (b) Snow depth during the critical period for tawny owl survival during 1981–2008 in Southern Finland. (c) Survival of grey and brown tawny owl colour morphs during 1981–2008. Grey tawny owls are denoted by grey circles and brown ones by red diamonds. Error bars are standard errors of the estimated survival and the lines are regression slopes based on the data. Figure 3: Survival of grey and brown tawny owls in relation to changes in snow depth. Survival estimates are based on averaging all candidate capture–mark–recapture models considering the effects of food supply (vole abundance), average snow depth and average temperature during a critical period in winter (see Supplementary Information ). Climatic data are derived from the database of the Finnish Meteorological Institute. ( a ) Survival of brown and grey tawny owl colour morphs in relation to snow depth. ( b ) Snow depth during the critical period for tawny owl survival during 1981–2008 in Southern Finland. ( c ) Survival of grey and brown tawny owl colour morphs during 1981–2008. Grey tawny owls are denoted by grey circles and brown ones by red diamonds. Error bars are standard errors of the estimated survival and the lines are regression slopes based on the data. Full size image Population-level response to climate-driven selection When selection on a heritable trait changes, a response in the composition of the population is expected [19] . We indeed found that the frequency of brown morphs increased markedly between 1981 and 2008. Compared with historical data, when on average one-third of the individuals were brown ( Fig. 4a ), we found that the brown morph rapidly increased in frequency especially during the last decade ( Fig. 4b ; binomial generalized linear model 1981–2008, year: b =0.050±0.009 s.e.m., z =5.66, N =28, P <0.0001). This phenotypic change was present also on a larger nationwide scale. In a time series of tawny owls captured, marked and colour scored (grey or brown) by ornithologists all over Finland between 1961 and 2008 ( N =3,239 observations), we found a steadily increasing frequency of the brown morph ( Fig. 4c , year: b =0.025±0.004 s.e.m., z =6.94, N =48, P <0.0001). Thus, the increase of the brown morph is a large scale phenomenon occurring all over Finland, involving thousands of individuals. Hence, this phenotypic change is unlikely to be caused by genetic drift, because drift is only a major force for changing allele frequencies in small populations. Given the strong genetic underpinning of tawny owl morphs (see above), we consider the observed phenotypic trend in the proportion of the brown morph as indicative for a shift in gene frequencies. Hence, we here document microevolution of tawny owl plumage colour. 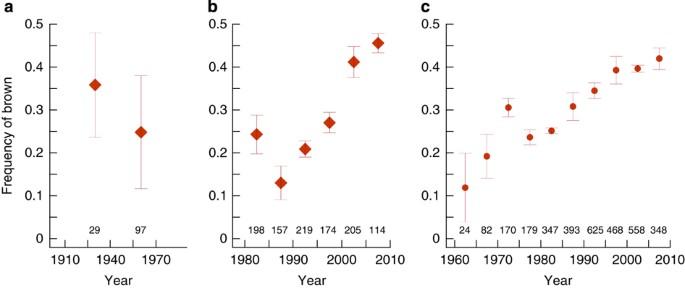Figure 4: Temporal changes in the frequency of the brown morph in Finland on different scales. (a) Historical data on colour morph frequencies in the early century (1911–1945) and mid-century (1946–1980) based on skins from the Zoological museum collection (University of Helsinki). Each symbol represents the mean frequencies of seven 5-year periods (± s.e.m.). (b) Frequency of the brown morph in the study population based on captured breeding birds between 1981 and 2008. Shown are mean annual frequencies of the brown morph in 5-year periods (±s.e.m.). (c) Nationwide population frequency of brown individuals based on all breeding birds ringed or recaptured by amateur ringers in Finland and colour scored as either grey or brown. Symbols are as inb. Total sample size is given along thexaxis. The method of scoring colour morphs inaandb(filled diamonds) differs from the method used inc(filled dots), such that the averages and slope of the trend are not directly comparable, although the direction is. Figure 4: Temporal changes in the frequency of the brown morph in Finland on different scales. ( a ) Historical data on colour morph frequencies in the early century (1911–1945) and mid-century (1946–1980) based on skins from the Zoological museum collection (University of Helsinki). Each symbol represents the mean frequencies of seven 5-year periods (± s.e.m.). ( b ) Frequency of the brown morph in the study population based on captured breeding birds between 1981 and 2008. Shown are mean annual frequencies of the brown morph in 5-year periods (±s.e.m.). ( c ) Nationwide population frequency of brown individuals based on all breeding birds ringed or recaptured by amateur ringers in Finland and colour scored as either grey or brown. Symbols are as in b . Total sample size is given along the x axis. The method of scoring colour morphs in a and b (filled diamonds) differs from the method used in c (filled dots), such that the averages and slope of the trend are not directly comparable, although the direction is. Full size image Apart from selection, immigration is an important population dynamical feature in our study population [24] . A proportional increase in immigrating brown morphs could account for the observed increase in their frequency in the population. To test the relative importance of morph-specific immigration, local recruitment and selection on the proportional increase of the brown morph, we categorized all breeding individuals into immigrants (first breeder that is unmarked or marked outside the study area), local recruits (first breeders marked as young) and old breeders (survivors from a previous breeding attempt). We then analysed the relative contribution of grey and brown survivors, immigrants and local recruits over time to the observed increase in the frequency of the brown morph. We found that the increase in frequency of the brown morph in the population was explained only by an increase in the number of brown survivors over time, and not by any other numeral trend (binomial generalized linear model: b =0.18±0.09 s.e.m., z =2.11, N= 28, P =0.035, Fig. 5 ). We used our observed parent–offspring inheritance pattern to retrospectively infer the morphs of offspring produced during the last three decades. There was no morph-specific temporal trend in reproductive success or recruitment rate ( Supplementary Information ), which illustrates that the increase in the proportion of brown morphs in the population is not driven by a change in productivity of the brown morph. Furthermore, we found no evidence for a phenotypically plastic within-individual colouration change as winter climate gets milder ( Supplementary Information ). We conclude that improved survival of brown adult tawny owls caused by warmer winters with less snow is the most likely candidate to drive the observed temporal increase in the brown morph. 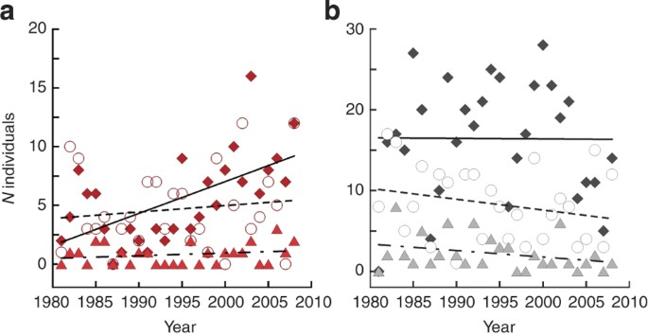Figure 5: Factors explaining the increase in the proportion of the brown morph in the study population. Number of brown (a) and grey (b) survivors (denoted by diamonds, solid line), immigrants (circles, dashed line) and recruits (triangles, dashed-dotted line) in the breeding population during the study period. Figure 5: Factors explaining the increase in the proportion of the brown morph in the study population. Number of brown ( a ) and grey ( b ) survivors (denoted by diamonds, solid line), immigrants (circles, dashed line) and recruits (triangles, dashed-dotted line) in the breeding population during the study period. Full size image Our study constitutes, to our knowledge, the first empirical evidence of climate-driven change in selection on a heritable trait. Work on climate change induced evolution typically concerns the documentation of temporal trends in traits that are assumed to be fitness-related (for example, phenology), possibly linked with an exploration of the genetic underpinning of such traits [3] . Even if a focal trait is heritable and selectively important, surprisingly few studies have asked whether climate change has actually altered the selective regime. Selection can be environmentally dependent and yet not change as climate changes [25] . Unless there is evidence that climate change drives an alteration in selection, it is potentially erroneous to attribute an observed temporal change in a trait (whether on the genetic or on the phenotypic level) to climate change, because a temporal trend can be caused also by other changes in the environment that occurred during the same time period. In this study, we show that a particularly powerful form of natural selection (survival selection on reproducing adults) on tawny owl colour polymorphism is driven by climatic conditions in early winter. Differential performance of contrasting morphs under variable environmental conditions lies at the heart of theory behind the evolution of genetic polymorphism [26] . There are three non-mutually exclusive explanations for why the brown tawny owl morph may be more sensitive to harsh winter conditions. First, colouration itself may be the target of selection; for example, predation on brown individuals may be more severe under snow-rich conditions. The main tawny owl predator, however, is the eagle owl Bubo bubo [27] , which is not a visual predator. Furthermore, the brown morph is in fact considered to be more cryptic [28] , although this need not hold under snow-rich conditions. Second, colouration may, through pleiotropic effect be associated with another property that is the real target of selection. Increasing evidence, both on molecular and individual level, suggests that the differential performance of morphs across environments can be caused by genetic covariation between colouration (melanization) and a physiological property, such as metabolism or immune function [14] , [18] , [29] , [30] , [31] , [32] . Third, pleiotropic effects between energy homoeostasis and melanin pigmentation can lead to differential predation pressure if the melanistic (brown) morph has higher energetic requirements and needs to forage more and thus becomes more susceptible to predation under harsh winter conditions. Additional research is needed in establishing the possible pleiotropic link between genes expressing colouration and physiological properties. Nevertheless, the observed pattern with an interaction between winter harshness and morph suggests that intrinsic differences between the morphs drive their propensity for survival. Our second main finding is a clear temporal shift towards a higher proportion of the brown morph in the population. In general, such a pattern is microevolution (change in allele frequencies driven by selection), genetic drift (stochastic change in allele frequency) or phenotypic plasticity (environmentally induced change in expressed phenotype) [3] . We show that the increase of the brown tawny owl morph occurs in a representative (nationwide) sample of the entire Finnish population of tawny owls (thousands of individuals), which makes it unlikely that random genetic drift drives this trend. The observed trend concerns phenotypes, but we here demonstrate that tawny owl morphs are under tight genetic control in a manner that is consistent with a one locus–two allele genetic architecture. In addition, we demonstrate that phenotypic plasticity does not explain the trend. We therefore believe that the increase in the proportion of brown tawny owls during the last two decades constitutes a microevolutionary change. A recent review [3] concluded that three study systems provide evidence for microevolutionary changes over time with a putative link to climate change. These are: a shift in the critical photoperiod that affects diapause in pitcher-plant mosquitoes [33] , shifts in the distribution of chromosomal arrangements and Adh alleles in Drosophila [4] , [5] , and quantitative genetic evidence that timing of breeding in red squirrels Tamiasciurus hudsonicus advanced in concert with climate warming [7] . For the first two examples, climate change could not be firmly established as the causal agent of the temporal change [3] . Recent developments in quantitative genetics [34] suggest that the last example is not as rigorous a demonstration of microevolution as initially suggested. We show that warming of winter climate leads to reduced selection against the brown morph, and we demonstrate that at the same time the frequency of the brown morph in the Finnish population increases to a level that is above the historic record of the species. Intuitively, a release of selection on a highly heritable trait should lead to a microevolutionary response, and we provide statistical evidence that selection (rather than immigration or local recruitment) indeed drives the observed increase in the frequency of the brown morph. On the other hand, our survival analysis does not show a selective advantage of the brown morph: survival during the last (warm) winters was approximately equal for the grey and brown morphs. Furthermore, the brown morph has no reproductive advantage. How can the frequency of the brown increase despite an absence of selective advantages? We believe that as yet unknown details of the genetics provide the link between the climate-driven change in selection and the observed increase in the frequency of the brown morph. In particular, we currently lack detailed quantitative understanding of how the selective mechanism operates on the genotypes. This is because if one accepts that morph inheritance patterns are caused by a one locus–two allele model with brown dominance over grey (as our findings suggest), there are two genotypes that produce a brown morph (heterozygous Bg and homozygous BB ), but we necessarily measure selection on these two combined (that is, morph-based). One possibility is that winter climate-driven selection against the heterozygote is less than selection against the homozygote. Indeed, if pleiotropic effects of the putative grey and brown colour genes indeed cause the differential survival of tawny owl morphs then a heterozygote brown individual may well perform differently than a homozygous brown individual. In the buzzard Buteo buteo , Mendelian inheritance of colour genes has been suggested to underlie the plumage colour polymorphism observed in that species with a selective advantage for the heterozygous morph [35] . From a population-genetic perspective, such a 'hidden' heterozygote advantage in combination with a temporal release of selection has the potential to explain both the maintenance of the brown morph in the population and the increase in frequency of the brown morph, despite the fact that selection continuously acts against the brown morph (model developed in Supplementary Information ). This hypothesis is testable once the molecular genetic basis of tawny owl plumage colour polymorphism has been clarified and selection on the genotypic level can be estimated. Our study demonstrates a climate change driven alteration of selection on a heritable trait coupled with a population-level evolutionary response; all of which are required for long-term survival of species. Because colour polymorphism is highly heritable, studies on these systems are likely to provide important benchmark insights in the effects of environmental change on population level changes, not only in terms of phenotypic changes [36] , but also in terms of changes in genetic diversity and the evolvability of organisms (see also Supplementary Information ) and changes in latitudinal distributions of morphs in colour polymorphic species [37] . Data sets Tawny owls were studied from 1981 to 2008 in a study area of about 250 km 2 in Southern Finland (60°15N′, 24°15E′). The study area is dominated by mixed forests, agricultural areas and small freshwater courses and was established in 1977–78. From 1980 onwards ∼ 125 nest boxes in suitable habitats were available for tawny owls to breed in. Considerable effort was put into finding the nests of all tawny owls in the study population by searching for natural nest sites and new boxes set up by private individuals in the approximate area where hooting individuals had been recorded earlier in spring and where a breeding thus was expected. The same monitoring scheme was used by K.A. and T.K. during all years and the effort remained similar in all years. The majority of all breeding male and female owls in the study population were caught, ringed and their reproductive output was measured. Plumage colouration was scored using a semi-continuous ordinal scale (range from 4 (grey) to 14 (reddish-brown)) on all breeding individuals on each encounter ( N =1116 records of 491 individuals) using a standardized and repeatable scoring that shows colouration is independent of age and sex [18] . Museum skin specimens collected by the public between 1915 and 1980 and stored by the Natural History Museum, University of Helsinki, ( N =126) were colour scored in the same way as in the study population. National level tawny owl colour morph data collected by ornithologists in Finland were obtained from the Finnish Ringing Centre. We extracted the data on all records of adult ringed and recaptured tawny owls in Finland to which colour morph (grey or brown) had been assigned during 1961–2008 (30% of all data, 3,194/10,601 records). Genetics. We used a REML linear mixed model ('animal model') to estimate heritability of plumage colouration. The additive genetic effects were estimated using pedigree-derived estimates of relatedness across all individuals [19] . We tested whether parent–offspring resemblance (83 nests with 318 offspring, data from 2006 to 2009) followed a purely additive genetic model, or a one locus–two allele model under Hardy–Weinberg equilibrium, in which either 'brown' or 'grey' were dominant over the other allele. Capture–mark–recapture modelling and model selection Survival of adult grey and brown tawny owls was estimated using capture–mark–recapture methodology on live encounters data (Cormack–Jolly–Seber model) of 1,065 observations of 466 tawny owls Supplementary Table S3 , using the programme MARK [38] . We used a sliding-window approach (all possible time windows between 5 and 44 days were considered) to find the relevant time period during which survival (full-time dependent CMR model, Φ ( t ) p ( t ) ) correlated best with climate (average temperature and snow depth). Annual survival of tawny owls was highly correlated with temperature and snow depth ( Supplementary Table S4 ). Measures of temperature and snow depth from the time window that correlated best with annual tawny owl survival were selected as covariates for further modelling ( Supplementary Table S4 ). We tested for the effects of real covariates by replacing the dummy variable 'time dependence ( t )' with interactions of colour morph and prey abundance (col*vole), temperature (col*temp) and snow depth (col*snow) in both survival (Φ) estimation as well as recapture ( p ). We applied model averaging [39] on the candidate models to get a more conservative estimate of Φ and p . Although averaging is performed over all candidate models, the weighting by QAIC model weights ensures that the information in the best fitting models contributes most. Further methodological details are provided in the Supplementary Methods . How to cite this article: Karell, P. et al . Climate change drives microevolution in a wild bird. Nat. Commun. 2:208 doi: 10.1038/ncomms1213 (2011).